Elastic anisotropy of experimental analogues of perovskite and post-perovskite help to interpret D′′ diversity Recent studies show that the D′′ layer, just above the Earth's core–mantle boundary, is composed of MgSiO 3 post-perovskite and has significant lateral inhomogeneity. Here we consider the D′′ diversity as related to the single-crystal elasticity of the post-perovskite phase. We measure the single-crystal elasticity of the perovskite Pbnm -CaIrO 3 and post-perovskite Cmcm -CaIrO 3 using inelastic X-ray scattering. These materials are structural analogues to same phases of MgSiO 3 . Our results show that Cmcm -CaIrO 3 is much more elastically anisotropic than Pbnm -CaIrO 3 , which offers an explanation for the enigmatic seismic wave velocity jump at the D′′ discontinuity. Considering the relation between lattice preferred orientation and seismic anisotropy in the D′′ layer, we suggest that the c axis of post-perovskite MgSiO 3 aligns vertically beneath the Circum-Pacific rim, and the b axis vertically beneath the Central Pacific. Since the discovery of the transition from perovskite (Pv) to post-perovskite (pPv) in MgSiO 3 (refs 1 , 2 ), pPv-MgSiO 3 has been considered to be a major component of the D′′ layer just above the core–mantle boundary (CMB). Seismological observations of the D′′ layer are difficult to interpret as they suggest both non-uniform response at the layer boundary and non-uniform anisotropy inside the layer [3] , [4] , [5] . With this background, elastic anisotropy or single-crystal elasticity of pPv-MgSiO 3 has been the focus of theoretical calculations [6] , [7] , [8] , [9] , [10] . However, no experimental data are available on the single-crystal elasticity of pPv-MgSiO 3 , because it is unstable at ambient pressure. Cmcm -CaIrO 3 or pPv-CaIrO 3 has been frequently selected as a representative analogue of pPv-MgSiO 3 (refs 11 , 12 , 13 ). According to the phase diagram [14] , pPv-CaIrO 3 is the stable phase at ambient conditions and Pv-CaIrO 3 is the high-temperature and low-pressure phase. Here we report the first experimental data on single-crystal elasticity of Pv and pPv structures in a homogeneous chemical composition of CaIrO 3 . 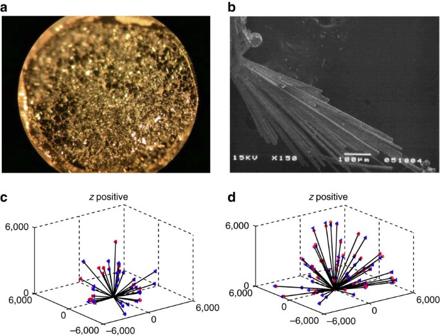Figure 1: Specimen and measurement data. Left and right columns refer toPbnm- andCmcm-CaIrO3, respectively. (a,b) Photographs of single crystals used. The horizontal edge lengths are ~5 mm and ~800 μm, respectively, foraandb. (c,d) Overall picture for the experimental data and analytical fitting. Black lines indicate the direction of wave propagation in the crystal, and blue triangles and red circles are experimental velocities and recalculated values after least-squares analysis. The vertical direction is positivezdirection, while horizontal leftward and rightward directions are positivexandydirections, respectively. Note that the difference between experimental and recalculated velocities is less than 5%. The misfit uniformly distributed indicates untwinned crystal specimens. Characterization of single-crystal specimen Figure 1a,b shows single crystals of Pv-CaIrO 3 and pPv-CaIrO 3 used in the present study. The Pv-CaIrO 3 sample was synthesized at 2 GPa and 1,450 °C for 15 h in a piston cylinder apparatus at Okayama University. We produced many grains with size of a few tens of microns, although most of them turned out to have multiple domains. We examined more than 20 grains using a four-circle X-ray diffractometer at Yamaguchi University and selected a quasi-single-domain crystal with size of ~20 μm. Its lattice constants were determined as a =5.3527(1), b =5.5969(5) and c =7.6804(6) Å, which yields density (ρ) of 8,091 kg m −3 . The pPv-CaIrO 3 sample was synthesized by slow cooling from 1,000 °C in CaCl 2 flux [15] . It had a pine-needle shape with length of a few 100 microns and width of a few 10s of microns. Its lattice constant and densities were respectively a =3.145(2), b =9.861(6), and c =7.297(5) Å, and ρ=8,211 kg m −3 , which are consistent with literature values [16] . Figure 1: Specimen and measurement data. Left and right columns refer to Pbnm - and Cmcm -CaIrO 3 , respectively. ( a , b ) Photographs of single crystals used. The horizontal edge lengths are ~5 mm and ~800 μm, respectively, for a and b . ( c , d ) Overall picture for the experimental data and analytical fitting. Black lines indicate the direction of wave propagation in the crystal, and blue triangles and red circles are experimental velocities and recalculated values after least-squares analysis. The vertical direction is positive z direction, while horizontal leftward and rightward directions are positive x and y directions, respectively. Note that the difference between experimental and recalculated velocities is less than 5%. The misfit uniformly distributed indicates untwinned crystal specimens. Full size image Inelastic X-ray scattering measurement and results Figure 1c,d compare experimental velocities obtained from the inelastic X-ray scattering (IXS) spectra with velocities calculated from the optimized elastic constants. The details of the IXS measurement are described in the Methods section for the measurement of IXS at SPring-8 BL35XU; one of the important advantages of IXS compared with Brillouin scattering is its geometrical freedom (see Supplementary Methods ). The analytical procedures for determining single-crystal elastic constants are described in the Methods section for data analysis for elastic constants. The measurement data are summarized in Supplementary Tables 1 and 2 . Table 1 summarizes the results of elastic constants and gives isotropic averages. The values are reasonably consistent with the theoretical results [17] except for a few discrepancies. The high-pressure phase of pPv-CaIrO 3 is less compressible than Pv-CaIrO 3 whereas the theoretical prediction suggests the opposite relation. In addition, isotropic averages of V P and V S are significantly larger for pPv-CaIrO 3 than for Pv-CaIrO 3 according to the present results. 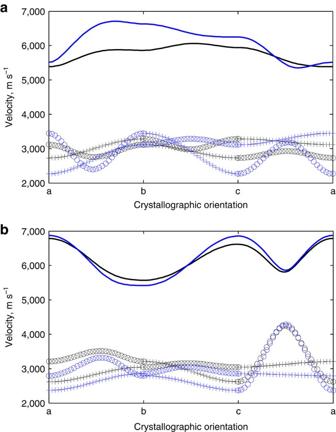Figure 2: Velocity surface ofPbnm- andCmcm-CaIrO3. Upper (a) and lower (b) plots correspond toPbnm- andCmcm-CaIrO3, respectively. Black lines are drawn for the present results, while blue lines are drawn for the results obtained by Tsuchiya and Tsuchiya17. Upper lines correspond to the P-wave velocity, and lower lines to the S-wave velocity. Open circles ‘o’ and crosses ‘+’ forVSspecify in-plane and out-of-plane particle motions. Figure 2 compares the present results and theoretical calculations for the velocity surfaces of Pv-CaIrO 3 and pPv-CaIrO 3 . We see fairly good agreement between the two results for pPv-CaIrO 3 , although we recognize significant differences between them for Pv-CaIrO 3 . 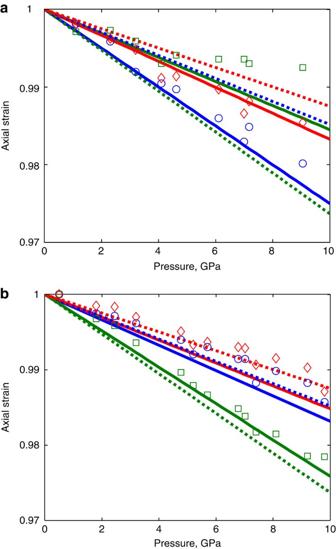Figure 3: Comparison of compression curves. Upper (a) and lower (b) plots correspond toPbnm- andCmcm-CaIrO3, respectively. The lattice constantsa,b, andcare shown in blue, green and red respectively. Solid and dotted lines are drawn for the present data and Tsuchiya’s theoretical data17, respectively, while symbols are the compression data. Figure 3 shows the compatibility of the elastic constants with compression data [18] . The present data are consistent with the compression data for Pv- and pPv-CaIrO 3 ; the theoretical result for Pv-CaIrO 3 , however, yields a different slope from the others. Table 1 Single-crystal elastic moduli of Pbnm - and Cmcm -CaIrO 3 . Full size table Figure 2: Velocity surface of Pbnm - and Cmcm -CaIrO 3 . Upper ( a ) and lower ( b ) plots correspond to Pbnm - and Cmcm -CaIrO 3 , respectively. Black lines are drawn for the present results, while blue lines are drawn for the results obtained by Tsuchiya and Tsuchiya [17] . Upper lines correspond to the P-wave velocity, and lower lines to the S-wave velocity. Open circles ‘o’ and crosses ‘+’ for V S specify in-plane and out-of-plane particle motions. Full size image Figure 3: Comparison of compression curves. Upper ( a ) and lower ( b ) plots correspond to Pbnm - and Cmcm -CaIrO 3 , respectively. The lattice constants a , b , and c are shown in blue, green and red respectively. Solid and dotted lines are drawn for the present data and Tsuchiya’s theoretical data [17] , respectively, while symbols are the compression data. Full size image 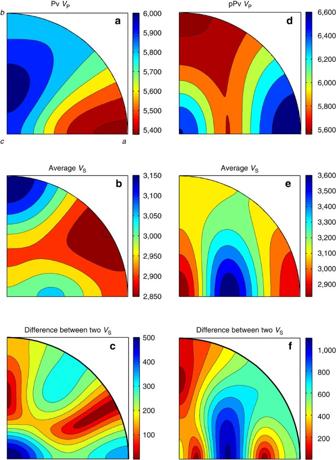Figure 4: Velocity surface of Pv- and pPv-CaIrO3. Stereo projections of elastic wave velocities for Pv- and pPv-CaIrO3based on the present results. The crystallographic directions,a,b, and,c, are identical in each plot as shown in (a). The unit of scale bars is m s−1. (a–c)VP, average of twoVSvalues, and difference between twoVSvalues, respectively, for Pv-CaIrO3. (d–f) Same asa,b, andcbut for pPv-CaIrO3. Figure 4 presents stereo projections of elastic wave velocities for Pv and pPv structures of CaIrO 3 . It shows that the ranges of variation of V P , the average of V S values, and the difference in V S values are ~600, ~300 and ~500 m s −1 for Pv-CaIrO 3 and ~1,000, ~800 and ~1,100 m s −1 , for pPv-CaIrO 3 , respectively. We see that pPv-CaIrO 3 has approximately double the anisotropy of Pv-CaIrO 3 in terms of the elastic wave velocity. For example, anisotropy in the polarization shear wave velocity is ~30% in pPv-CaIrO 3 while it is only ~15% in Pv-CaIrO 3 . Figure 4: Velocity surface of Pv- and pPv-CaIrO 3 . Stereo projections of elastic wave velocities for Pv- and pPv-CaIrO 3 based on the present results. The crystallographic directions, a , b , and, c , are identical in each plot as shown in ( a ). The unit of scale bars is m s −1 . ( a – c ) V P , average of two V S values, and difference between two V S values, respectively, for Pv-CaIrO 3 . ( d – f ) Same as a , b , and c but for pPv-CaIrO 3 . Full size image From Fig. 4d,e for pPv phase, the b axis is found to be the direction of the lowest V P , while the highest V s is between the a and c axes. These pronounced features of the pPv elasticity are understandable as alternate stacking of compliant and stiff layers perpendicular to the b axis; the stiff layer has the largest shear wave constant and lowest longitudinal wave constant between a and c axes. We recognize similarity between a and c axes in pPv-CaIrO 3 elasticity, while the a axis is slightly stiffer than the c axis in terms of both longitudinal and shear wave constants. The elasticity of Pv-CaIrO 3 resembles that of Pv-MgSiO 3 under lower-mantle conditions more than under ambient conditions ( Fig. 5 ). Elasticity of Pv- and pPv-CaIrO 3 under ambient conditions seems to be a good indicator of that of Pv- and pPv-MgSiO 3 under lowermost mantle conditions; a conversion factor of 2.2–2.4 is found between them. 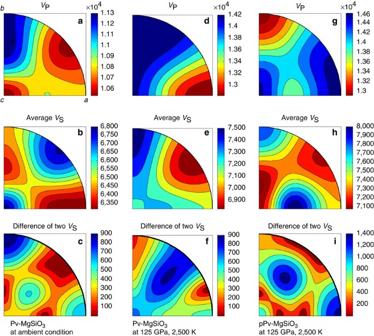Figure 5: Stereo projections of elastic wave velocities for Pv- and pPv-MgSiO3. The crystallographic directions,a,b, and,c, are identical in each plot as shown in (a). The unit of scale bars is m s−1, although a factor of 104should be multiplied forVP. (a–c)VP, average of twoVSvalues, and difference between twoVSvalues, respectively, for Pv-MgSiO3under ambient conditions. (d–f) and (g–i) Same asa,b, andcbut for Pv-MgSiO3and pPv-MgSiO3at 125 GPa and 2,500 K10, respectively. Figure 5: Stereo projections of elastic wave velocities for Pv- and pPv-MgSiO 3 . The crystallographic directions, a , b , and, c , are identical in each plot as shown in ( a ). The unit of scale bars is m s −1 , although a factor of 10 4 should be multiplied for V P . ( a – c ) V P , average of two V S values, and difference between two V S values, respectively, for Pv-MgSiO 3 under ambient conditions. ( d – f ) and ( g – i ) Same as a , b , and c but for Pv-MgSiO 3 and pPv-MgSiO 3 at 125 GPa and 2,500 K [10] , respectively. Full size image We interpret the D′′ diversity observed seismologically in terms of the single-crystal elasticity of Pv and pPv-CaIrO 3 . Significant anisotropy of the seismic wave velocity has been observed in the D′′ layer, while the lower mantle above the D′′ layer is nearly isotropic with a high degree of confidence [19] . Therefore, we plotted the velocity difference between anisotropic pPv and isotropic Pv both for CaIrO 3 under ambient conditions and MgSiO 3 under mantle conditions ( Fig. 6 ). From the plots for V P and slower V S , we see that any velocity change over the D′′ discontinuity is possible both for P and S waves depending on the lattice preferred orientation (LPO) characteristics of the pPv phase. 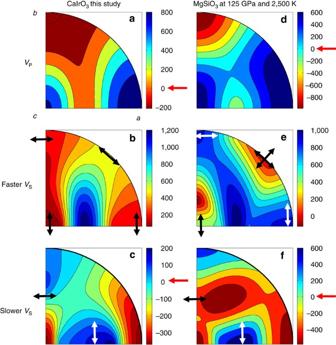Figure 6: Velocity difference between anisotropic pPv and isotropic Pv. The left column presents the results for CaIrO3in the present study, while the right column presents the theoretical calculation for MgSiO3at 125 GPa and 2,500 K10. We recognize common characteristics among the plots for the two materials. Isotropic P-wave velocities of Pv are 5,774 and 13,900 m s−1and S-wave velocities are 2,975 and 7,200 m s−1for CaIrO3and MgSiO3, respectively. The red arrows beside the scale bars highlight the origin of each scale bar, where the velocities of the two phases are the same. Typical polarizations of the S wave are shown by arrows in the S-wave plots. The crystallographic axes are identical for all plots as shown in plota. In the stereo projections, the propagating waves in thea–bandc–aplanes are shown along the quarter arc and the bottom edge, respectively. Note that the two polarization arrows in plotebetweenaandbaxes suggest that the two S-wave velocities are nearly the same, as shown inFig. 7. Figure 6: Velocity difference between anisotropic pPv and isotropic Pv. The left column presents the results for CaIrO 3 in the present study, while the right column presents the theoretical calculation for MgSiO 3 at 125 GPa and 2,500 K [10] . We recognize common characteristics among the plots for the two materials. Isotropic P-wave velocities of Pv are 5,774 and 13,900 m s −1 and S-wave velocities are 2,975 and 7,200 m s −1 for CaIrO 3 and MgSiO 3 , respectively. The red arrows beside the scale bars highlight the origin of each scale bar, where the velocities of the two phases are the same. Typical polarizations of the S wave are shown by arrows in the S-wave plots. The crystallographic axes are identical for all plots as shown in plot a . In the stereo projections, the propagating waves in the a–b and c–a planes are shown along the quarter arc and the bottom edge, respectively. Note that the two polarization arrows in plot e between a and b axes suggest that the two S-wave velocities are nearly the same, as shown in Fig. 7 . Full size image The seismic wave phases used in the D′′ study (S, ScS, Sdiff) travel nearly horizontally in the D′′ layer [4] . Therefore, the two polarized S waves are classified as SH and SV, whose polarizations are in the horizontal and vertical directions, respectively. In seismological study, vertically transverse isotropy (VTI) and the tilted transverse isotropy have been assumed to explain S-wave polarization anisotropy in the D′′ layer [4] . According to seismological studies, the region of the Circum-Pacific rim is interpreted as having VTI with V SH > V SV , while the region of the Central Pacific has complicated VTI without any fixed relation between V SH and V SV [4] . Polarization anisotropy is not recognized beneath the Atlantic Ocean, or the region is considered as having VTI with V SH ≈ V SV . On the other hand, from the polarization pattern in the a–b plane of the faster V S plot ( Figs 2b and 7 ), we can expect that V SH > V SV in the D′′ layer if the c axis of pPv aligns vertically. Similarly, if the b axis aligns vertically, the magnitude relation between V SH and V SV can be complicated. 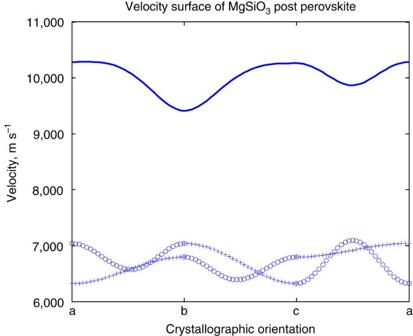Figure 7: Velocity surfaces of pPv-MgSiO3at 125 GPa and 2,500 K. Blue lines are used to specify theoretical results similar toFig. 2a,b. The upper line is the P-wave velocity and the lower lines are the S-wave velocities. Open circles ‘o’ and crosses ‘+’ forVSspecify in-plane and out-of-plane particle motions. Figure 7: Velocity surfaces of pPv-MgSiO 3 at 125 GPa and 2,500 K. Blue lines are used to specify theoretical results similar to Fig. 2a,b . The upper line is the P-wave velocity and the lower lines are the S-wave velocities. Open circles ‘o’ and crosses ‘+’ for V S specify in-plane and out-of-plane particle motions. Full size image We can summarize the above conclusion in an alternative way: For the c axis vertical case, horizontal wave propagation directions lie in the a–b plane, for which the in-plane shear mode (SH) has consistently higher wave speeds ( Figs 2b and 7 ). If instead the b axis is vertical, horizontal wave propagation directions lie in the a–c plane, for which neither the in-plane (SH) nor the out-of-plane (SV) is consistently faster for all such propagation directions ( Figs 2b and 7 ). The dominant slip system of pPv-CaIrO 3 was determined as [100](010) from shear deformation experiments [11] . Since the slip system of pPv-MgSiO 3 has not yet been determined, we assumed that it is similar to that of pPv-CaIrO 3 [11] . This assumption leads to LPO of pPv-MgSiO 3 , in which the b axis aligns vertically along the lateral flow in the D′′ layer. The LPO pattern is consistent with the complicated polarization S-wave anisotropy beneath the Central Pacific ( Figs 2b and 7 ). Although the texture development during Pv–pPv transition in MgSiO 3 has not yet been clarified, we expect the c axis alignment of pPv-MgSiO 3 immediately after the phase transition from Pv-MgSiO 3 from analogy with the case for MgGeO 3 (ref. 20 ). If the c axis aligns vertically, we expect VTI with V SH > V SV, which is consistent with the seismic feature beneath the Circum-Pacific rim. Employing this conceptual scheme, we evaluated the feasibility of the LPO model of pPv in the D′′ layer. The volume ratio between (Mg, Fe)SiO 3 Pv and (Mg, Fe)O ferropericlase (Fp) is 0.67:0.33 for the lower mantle [21] . We also used this ratio for (Mg, Fe)SiO 3 pPv and Fp in the D′′ layer. This means that the anisotropy resulting from pPv LPO should be weakened by approximately two-thirds in the D′′ layer assuming isotropy of Fp. The observed polarization anisotropy of the S-wave velocity is ~3% at most [4] . Therefore, pPv in the D′′ layer is expected ~4.5% anisotropy to account ~3% anisotropy observed in the D” layer. This requirement is easily satisfied by partial LPO of pPv ( Table 2 ). Table 2 Characteristic velocities for crystals of post-perovskite structure. 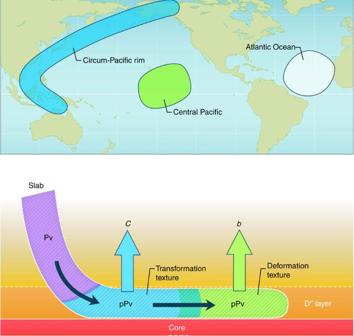Figure 8: Schematic illustration of the LPO of pPv-MgSiO3in the D′′ layer. From a mineral physics viewpoint, the Pv slab (purple region) transforms to pPv (light blue region) and the pPv slab then moves along the path of mantle convection with deformation (light-green region). In contrast, from seismic observation, the region of the Circum-Pacific rim has VTI anisotropy ofVSH>VSV, while the region of the Central Pacific has complicated VTI with any magnitude relation; that is,VSH>VSV,VSH<VSVorVSH≈VSV. The region of the Atlantic Ocean (white circle) has VTI withVSH≈VSV, suggesting isotropy or negligible LPO of pPv-MgSiO3. The speculated aligned axes of pPv LPO are shown by arrows for each region; the verticalcaxis beneath the Circum-Pacific rim and the verticalbaxis beneath the Central Pacific. Full size table Figure 8 summarizes the present idea for seismic anisotropy and LPO structure in the D′′ layer. The VTI of the vertical c axis and that of the vertical b axis can be interpreted as transformation LPO and deformation LPO, respectively. It is noted that isotropic pPv-MgSiO 3 is a reasonable interpretation for the seismic feature beneath the Atlantic Ocean; an alternative interpretation may be the VTI of the vertical a axis because of less lateral polarization anisotropy than in other cases ( Table 2 ). The difference between beneath the Pacific and Atlantic may be attributed to differences in temperature, chemical composition and strain rate. The proposed LPO behaviour for pPv-MgSiO 3 obtained from the present mineral physics perspective is consistent with seismic observation. Figure 8: Schematic illustration of the LPO of pPv-MgSiO 3 in the D′′ layer. From a mineral physics viewpoint, the Pv slab (purple region) transforms to pPv (light blue region) and the pPv slab then moves along the path of mantle convection with deformation (light-green region). In contrast, from seismic observation, the region of the Circum-Pacific rim has VTI anisotropy of V SH > V SV , while the region of the Central Pacific has complicated VTI with any magnitude relation; that is, V SH > V SV , V SH < V SV or V SH ≈ V SV . The region of the Atlantic Ocean (white circle) has VTI with V SH ≈ V SV , suggesting isotropy or negligible LPO of pPv-MgSiO 3 . The speculated aligned axes of pPv LPO are shown by arrows for each region; the vertical c axis beneath the Circum-Pacific rim and the vertical b axis beneath the Central Pacific. Full size image To summarize, we presented a new data set of Pv and pPv-CaIrO 3 single-crystal elasticity by means of IXS at SPring-8. We used the present results to interpret seismic wave anisotropy in the D′′ layer, and proposed a model of pPv LPO in the D′′ layer consistent with seismic observations and mineral physics experiments on analogue materials. The present model may allow sophisticated discussion of global mantle convection, which is triggered by heating at the core–mantle boundary and modulated by lateral flow in the D′′ layer. Measurement of IXS at SPring-8 BL35XU The small size and black colour of the present samples limit the techniques that can be used to investigate the elastic properties. In particular, the crystal sizes are too small to employ GHz ultrasonic methods [22] or resonant ultrasound spectroscopy [23] , where both need crystals larger than 100 μm. In addition, the crystal opacity makes it difficult to apply Brillouin scattering. Therefore, IXS with an X-ray beam diameter of ~70 μm was employed. Each specimen was attached to glass fibres (~100 μm in diameter) using manicure resin and mounted on the four-circle goniometer installed at BL35XU of SPring-8 (ref. 24 ). The incident X-ray beam energy was 17.794 and 21.747 keV for Pbnm -CaIrO 3 and Cmcm -CaIrO 3 measurements, respectively. The IXS technique [25] , [26] allows us to determine the elastic properties of a material by measuring the energies of acoustic longitudinal and shear phonon modes. When this information is combined with the precise reciprocal space position (momentum transfer) for each measurement, we can determine the sound velocity [27] , [28] . If measurements are made in many different directions, the velocity information can be combined with the density, allowing all the elastic constants of a material to be determined. In the present work, the two-dimensional, 4 × 3, analyser array of BL35XU is especially advantageous as it allows access to 12 different directions of momentum transfer simultaneously. The IXS is applicable on opaque materials; it is the most important advantage of IXS against Brillouin scattering. Further characteristics and procedures of the IXS measurements are summarized in Supplementary Figs 1–5 . Data analysis for elastic constants A least-squares fit to Christoffel equation was then used to determine the elastic constants [29] . Pv-CaIrO 3 and pPv-CaIrO 3 have orthorhombic symmetry and thus nine independent elastic constants. The six diagonal elastic constants ( C 11 , C 22 , C 33 , C 44 , C 55 , C 66 ) is related to nearly independent phonon modes propagating along crystallographic axes, while the three off-diagonal constants ( C 12 , C 23 , C 31 ) can be determined from combination of a few measurements. We carefully planned the measurement to acquire sufficient data to constrain all nine elastic constants. Using the analyser array, we obtained ~40 and ~60 mode energies for Pv-CaIrO 3 and pPv-CaIrO 3 , respectively. How to cite this article: Yoneda, A. et al. Elastic anisotropy of experimental analogues of perovskite and post-perovskite help to interpret D′′ diversity. Nat. Commun. 5:3453 doi: 10.1038/ncomms4453 (2014).